Enantioselective synthesis of helical polydiacetylene by application of linearly polarized light and magnetic field Magnetic optical activity, which can occur in all media and is induced by longitudinal magnetic field, causes the difference in absorption coefficients of left and right circularly polarized light and has the potential for magnetically induced enantioselectivity in chemical reactions. Compared with the well-established technique with circularly polarized light, there are few reports on the production of helical conjugated polymers in a photochemical reaction based on above magnetochiral anisotropy mechanism. Herein, we demonstrate experimentally that the enantioselective polymerization of diacetylene derivative can be achieved in the liquid crystal phase by application of linearly polarized light under a parallel or antiparallel magnetic field. The screw direction of predominant helical polydiacetylene chain can be rigorously controlled with the relative orientation of linearly polarized light and the magnetic field. Moreover, the prepared helical polydiacetylene assemblies can serve as a direct visual probe for the enantioselective recognition of D - or L -lysine. Symmetry breaking, leading to a specific handedness (left or right) of biological structure, is one of the most fascinating phenomena in nature [1] , [2] . In particular, the introduction of chiral nanostructure into conjugated polymer materials is expected to induce novel optical, electrical and magnetic properties, and tremendous potential for a wide variety of applications, such as organic devices with special electromagnetic functions and chirality sensing [3] . In the past decades, various helical conjugated polymers materials, including polythiophene [4] , polypyrrole [5] , polyaniline [6] and polydiacetylene (PDA) [7] have been synthesized through asymmetric polymerization, which can be proceeded if chiral monomers, dopants or catalysts are involved, or if some external chiral influence is present. One such external influence is circularly polarized light (CPL), which is inherently chiral and has been regarded as one source for the origin of homochirality in nature [8] . Left- and right-handed CPL have been used to induce the enantioselective photodecomposition of chiral organic compounds; however, only a small enantiomeric excess (<4%) could be obtained due to their very small anisotropy ( g ) factors [9] , [10] . Recently, Professor Iwamoto and our group demonstrated the synthesis of helical PDA through asymmetric polymerization with CPL [11] . Namely, left- or right-handed CPL irradiation yielded opposite helical polymers. The interaction between the CPL and the diacetylene (DA) dimer was assumed to play a key role in the enantioselective synthesis of helical PDA. Compared with the well-established technique using CPL, the effect on linearly polarized light (LPL) irradiation is usually interpreted as an instrumental artifact that arises from the combination of linear dichroism and birefringence of the aligned polymer chain [12] . However, induced by the longitudinal magnetic field, magnetochiral dichroism arises from the difference in absorption coefficients of left and right CPL [13] . By a similar mechanism, one can expect enantioselectivity in asymmetric chemical reactions with LPL under a magnetic field owing to magnetochiral dichroism [14] . Rikken and Raupach [15] have used above magnetochiral dichroism to favour the production of one enantiomer in a photochemical reaction. They used the chiral Cr(III) tris-oxalato complex, and showed that a small excess of one enantiomer was produced and maintained in the presence of an unpolarized laser beam travelling parallel to a static magnetic field. However, to the best of our knowledge, attempts to synthesize helical conjugated polymer based on above magnetochiral dichroism mechanism, especially from achiral monomer, have not been described to date [16] . Here, we demonstrate experimentally that the enantioselective polymerization of disc-shaped DA derivative can be achieved in the liquid crystal (LC) phase by application of LPL under a parallel or antiparallel magnetic field. The screw direction of predominant helical PDA chain can be controlled with the relative orientation of LPL and the magnetic field. Synthesis of helical PDA with LPL under a magnetic field Previously, we reported that the asymmetric polymerization of disc-shaped DA derivative ( Supplementary Fig. 1 ) could be realized on CPL irradiation in LC phase [17] , which could effectively provide chiral order in the chain propagating process. On the basis of a similar mechanism, we would expect to utilize magnetochiral dichroism to realize the enantioselective polymerization of DA units in the LC phase when one-sidedly irradiating above disc-shaped DA derivative under a static magnetic field parallel or antiparallel to the irradiation direction of LPL. The asymmetric photopolymerization reactions were carried out using the apparatus as shown in Fig. 1a . Photopolymerization reactions of DA units in the LC phase (at 47 °C) were performed by LPL under different magnetic field conditions (zero magnetic field, magnetic field perpendicular or parallel to the beam of LPL, respectively). After polymerization, all samples turned blue and exhibited typical intense absorption maximum at about 640 and 580 nm, confirming the formation of PDA chains ( Supplementary Fig. 2 ). The fractional conversion value for DA monomers in all samples was about 0.31. When above films were subjected to circular dichroism (CD) characterization, it was interesting to note that obvious CD signals (a positive and negative Cotton effect appeared at 550 and 670 nm with a crossover at 640 nm) could be observed at the corresponding absorption band for PDA backbone ( Fig. 1b ). To investigate the origin of the CD signal, measurements were carried out by rotating the sample about the normal of the films ( Supplementary Fig. 3 ). As in the case of zero magnetic field or the magnetic field perpendicular to the beam of LPL, only weak CD signal could be observed. The signal intensity drastically changed with the rotation angle, thus indicating that linear dichroism is the main origin of CD signals ( Supplementary Fig. 3a,b ). In contrast, in the case of the magnetic field parallel to the irradiation direction of LPL, the variation of the CD signal at all rotation angles was marginal compared with the intense CD signal, thus confirming that the main origin of CD signals should be the helix formation of PDA chains. To further confirm the origin and stability of CD signals, all samples were heated to 80 °C for 10 min and all of them turned red and exhibited typical intense absorption maximum at about 500 and 540 nm due to the thermochromic phase transition of PDA chains ( Supplementary Fig. 4a ). The samples, derived from the zero magnetic field or the magnetic field perpendicular to the irradiation direction of LPL, underwent CD signals erased during annealing treatment ( Supplementary Fig. 4b,c ). In contrast, in the case of the magnetic field parallel to the beam of LPL, CD signal was maintained, but showed a corresponding blue shift as that of the ultraviolet (UV) absorption band during the annealing process ( Supplementary Fig. 4d ) [18] . Moreover, 1,3,5-tris(1-alkyl-1 H -1,2,3-triazol-4-yl) benzene (TTB) cores could be further removed from the hydrogen-bonding (HB) complex on exposure to NH 3 gas [19] and then extraction with CHCl 3 ( Supplementary Fig. 5 ). However, CD signals for PDA chains were still maintained for the sample derived from the magnetic field parallel to the beam of LPL. 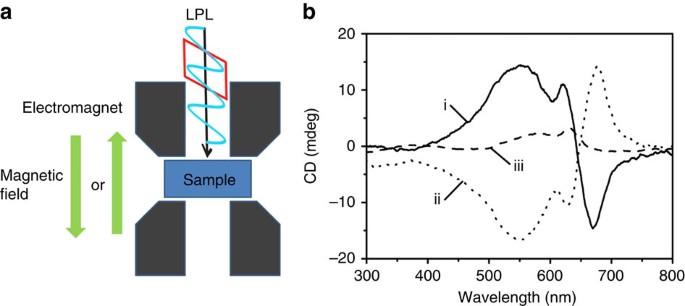Figure 1: Experimental set-up and CD spectra. (a) Experimental set-up for the enantioselective synthesis of helical PDA by application of LPL and magnetic field. (b) CD spectra of PDA films polymerized by application of LPL irradiation (10 mW cm−2) and the magnetic field (0.5 T): (i) parallel or (ii) antiparallel to the beam of LPL and (iii) with zero magnetic field. Figure 1: Experimental set-up and CD spectra. ( a ) Experimental set-up for the enantioselective synthesis of helical PDA by application of LPL and magnetic field. ( b ) CD spectra of PDA films polymerized by application of LPL irradiation (10 mW cm −2 ) and the magnetic field (0.5 T): (i) parallel or (ii) antiparallel to the beam of LPL and (iii) with zero magnetic field. Full size image Transmission electron microscopy characterization was carried out to investigate the morphology of the sample prepared by application of LPL irradiation in a parallel or antiparallel magnetic field ( Supplementary Fig. 6 ). The thus-formed predominant left-handed and right-handed helical PDA assemblies confirmed that photopolymerization of DA assemblies by application of LPL and magnetic field can be enantioselective. Significant CD signals with mutual mirror images were observed for the samples prepared by application of LPL and the magnetic field parallel or antiparallel to the irradiation direction (as shown in Fig. 1b ). The induced chiral excess was quantitatively characterized through second-harmonic generation (SHG) combined with linear dichroism (SHG-LD) method [20] , [21] , [22] . The typical polarization dependence curves of SH intensity from PDA films polymerized by application of LPL irradiation (10 mW cm −2 ) in a parallel magnetic field (0.5 T) were shown in Supplementary Fig. 7 . A significant difference in SH intensities at incident polarization angles of ±45° was actually observed, indicating the excess of the induced chirality. The values of DCE for the samples polymerized by application of LPL irradiation (10 mW cm −2 ) in a parallel or antiparallel magnetic field (0.5 T) were calculated to be 0.11±0.04 and −0.12±0.06, respectively. All above results indicated that photopolymerization of DA assemblies by application of LPL and magnetic field can be enantioselective, and the screw direction of the predominant helical PDA chain can be rigorously controlled with the relative orientation of LPL and the magnetic field. To further evaluate the degree of CD, we defined the absorption dissymmetry factor ( g ) as g =( ε L − ε R )/[( ε L + ε R )/2]=Δ ε / ε , where | g |<2 (ref. 23 ). The ε L and ε R were defined as the absorption coefficients of left- and right-handed polarized light, respectively. As shown in Supplementary Fig. 8 (refs 24 , 25 ), the samples under the magnetic field parallel or antiparallel to the irradiation direction of LPL clearly exhibited opposite g -factor values at the corresponding absorption band for PDA chains. In the case of magnetic field parallel or antiparallel to the irradiation direction of LPL, the absolute values of g -factor increased with the increasing intensity of the magnetic field, and a strictly linear relationship between the g -factor value and the magnetic field intensity B could be obtained ( Fig. 2a ), giving g / B =7.5 × 10 −4 T −1 . Besides, the g value hardly changed, although the polarizer rotation angle of LPL varied from 0 to 360° ( Fig. 2b ), indicating that the g -factor value was independent of the polarization state of the LPL. Moreover, the values of DCE for the samples polymerized by application of LPL irradiation (10 mW cm −2 ) in a parallel magnetic field (0.1, 0.3, 0.5 and 0.9 T) were calculated to be 0.03±0.02, 0.07±0.04, 0.11±0.04 and 0.15±0.05, respectively. The DCE values increased with the increase of the magnetic field intensity, but exhibited independent of the polarization state of the LPL. These results were in full agreement with the properties of the magnetochiral anisotropy, and proved that polymerization of DA units could be enantioselective. All above results confirmed that magnetochiral dichroism could be utilized to realize the enantioselective polymerization of DA units by application of LPL and magnetic field parallel or antiparallel to the irradiation direction of LPL. 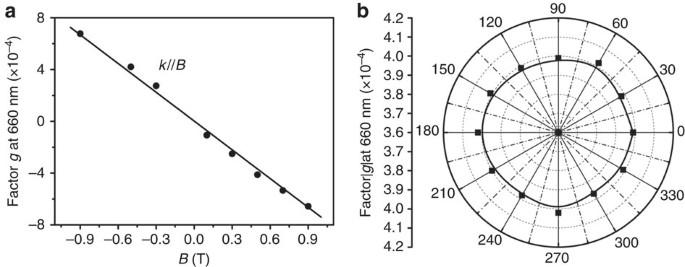Figure 2: Results of asymmetric photopolymerization with LPL under a magnetic field. (a) Theg-factor value obtained after irradiation with LPL (10 mW cm−2) for 3 min as a function of magnetic field intensity, with an irradiation direction k either parallel or antiparallel to the magnetic fieldB. (b) Theg-factor value obtained after irradiation with LPL (10 mW cm−2) for 3 min as a function of the polarizer rotation angle, with an irradiation direction k parallel to the magnetic fieldB(0.5 T). Figure 2: Results of asymmetric photopolymerization with LPL under a magnetic field. ( a ) The g -factor value obtained after irradiation with LPL (10 mW cm −2 ) for 3 min as a function of magnetic field intensity, with an irradiation direction k either parallel or antiparallel to the magnetic field B . ( b ) The g -factor value obtained after irradiation with LPL (10 mW cm −2 ) for 3 min as a function of the polarizer rotation angle, with an irradiation direction k parallel to the magnetic field B (0.5 T). Full size image Asymmetric polymerization mechanism As mentioned above, the helical PDA chains exhibited a typical g -factor extremum at 660 nm; therefore, it was reasonable to use the chronological development of the g -factor extremum to evaluate the enantioselective polymerization kinetics for the helical PDA chains with LPL under a parallel magnetic field. The kinetics curves clearly showed that the enantioselective polymerization process could also be described as a first order reaction (as shown in Fig. 3a ). The rate constant k 1 was determined to be 2.2 × 10 −2 s −1 with the magnetic field intensity maintained at 0.5 T and the intensity of LPL at 10 mW cm −2 . To further investigate the asymmetric polymerization mechanism, the kinetics constant k 1 was explored as a function of the light intensity of LPL, with the magnetic field (0.5 T) parallel to the irradiation direction. These results are plotted in Fig. 3b on a dual logarithmic scale. As can be seen, the asymmetric polymerization kinetics constant k 1 exhibited quadratic dependence on the light intensity of LPL, where the slop of the plots was about 2. All above results revealed that the formation mechanism of the helical PDA chains may involve biradical mechanism (the biradical dimer acted as the initiator in the DA polymerization process [26] ) as the primary species, similar as that on irradiation with CPL [27] . 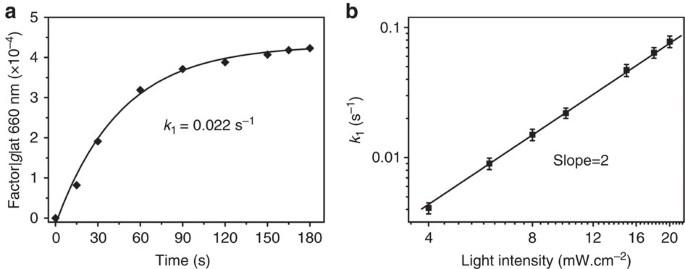Figure 3: Asymmetric polymerization kinetics. (a) Time-resolved development of the absolute value ofg-factor extremum at 660 nm on LPL irradiation (10 mW cm−2) with the magnetic field (0.5 T) parallel to the irradiation direction. (b) The dependence of the asymmetric polymerization kinetics constantk1on the light intensity of the LPL. Figure 3: Asymmetric polymerization kinetics. ( a ) Time-resolved development of the absolute value of g -factor extremum at 660 nm on LPL irradiation (10 mW cm −2 ) with the magnetic field (0.5 T) parallel to the irradiation direction. ( b ) The dependence of the asymmetric polymerization kinetics constant k 1 on the light intensity of the LPL. Full size image It has been reported that the photoinitiation of polymerization reaction depends on the excitation of DA monomers. On LPL irradiation in a parallel or antiparallel magnetic field, DA monomers preferentially absorbed one-handed circularly polarized component due to the magnetochiral dichroism effect, producing an excess of one-handed helical PDA oligomer chain. The thus-formed helical oligomer radical might be aligned in a suitable orientation and react more often with the neighbour DA monomer, eventually resulted in the formation of helical PDA chains predominantly in one chiral state. On the basis of the above discussion, the formation mechanism of the helical PDA chains by application of LPL and the magnetic field was illustrated in Fig. 4 . 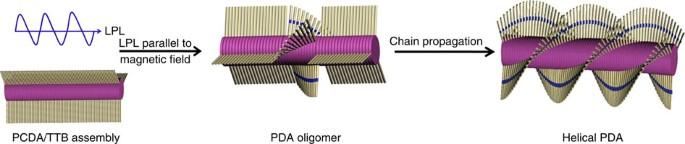Figure 4: Possible helix formation mechanism. Scheme forasymmetric polymerization mechanism for the HB complex samples prepared by application of LPL and the magnetic field parallel to the irradiation direction. Figure 4: Possible helix formation mechanism. Scheme forasymmetric polymerization mechanism for the HB complex samples prepared by application of LPL and the magnetic field parallel to the irradiation direction. Full size image Discrimination of amino acid enantiomers Enantioselective recognition of chiral molecules has attracted increasing interest since the two enantiomers of a chiral compound generally have different biological activities, especially in biomedical and pharmaceutical analysis [28] . The straight-forward and direct visual discrimination of chiral enantiomers still remains a major challenge in the design of chiral molecular sensors [29] . As mentioned above, left- or right-handed helical PDA assemblies could be prepared by application of LPL and the magnetic field. It is anticipated that the above helical PDA assemblies could be applied for the direct visual enantioselective recognition of chiral amino acids due to the destruction of HB interactions between TTB core and the peripheral helical PDA chains by basic amino acid [19] . Discrimination properties of above helical PDA assemblies were investigated by UV absorption and CD characterization. When above prepared left-handed helical PDA assemblies films was immersed into a cell with 5 ml aqueous solution of L -lysine (20 mg ml −1 ) for 2 h, an appreciable blue-to-red colour change could be observed. In the meantime, the absorbance at 580 and 640 nm reduced and new absorbance emerged at 500 and 540 nm ( Fig. 5a ). To evaluate this blue-to-red transition, we defined the colorimetric response (CR) as the relative change in ‘percent blue’ [30] . The initial percent blue, PB 0 is defined as PB 0 = A blue /[ A blue + A red ] × 100%, where A is the absorbance at either the ‘blue’ component in the UV–visible spectrum (640 nm) or the ‘red’ component (540 nm). The CR characterized the percent conversions to the red phase: CR=[PB 0 −PB 1 ]/PB 0 × 100%, where PB 1 is the final percent blue after immersion into the amino acid solutions. It revealed that on immersion into the L -lysine solution, the CR value for the left-handed helical PDA assemblies dramatically increased. However, no obvious colour or spectra changes could be detected when above sample was immersed into the D -lysine solution at the same concentration. CD characterization gave similar results, as shown in Supplementary Fig. 9 . Most interestingly, opposite recognition behaviour was observed for the right-handed helical PDA assemblies. Namely, when immersed into the D -lysine solution, the right-handed helical PDA assemblies exhibited obvious colour change and the CR value dramatically increased, while no obvious colour or spectra changes could be detected for the left-handed helical PDA assemblies ( Fig. 5b ). 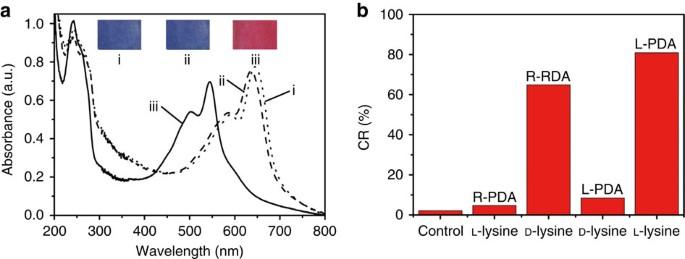Figure 5: UV–visible spectra and CR values. (a) UV–visible absorption spectra of the prepared left-handed PDA assemblies: (i) before treatment, immersed into (ii)D-lysine or (iii)L-lysine solution. The insert exhibits corresponding colour changes. (b) The CR value of the left- and right-handed PDA assemblies on response toD-lysine orL-lysine, respectively. Figure 5: UV–visible spectra and CR values. ( a ) UV–visible absorption spectra of the prepared left-handed PDA assemblies: (i) before treatment, immersed into (ii) D -lysine or (iii) L -lysine solution. The insert exhibits corresponding colour changes. ( b ) The CR value of the left- and right-handed PDA assemblies on response to D -lysine or L -lysine, respectively. Full size image The above-mentioned results motivated us to examine the CR values for the left-handed helical PDA assemblies immersed into the mixture solution of L - and D -lysine with various ratios (the total concentration of lysine isomers mixture was kept at 20 mg ml −1 ). As shown in Supplementary Fig. 10 , the CR value increased with a higher fraction of L -lysine. All above results confirmed that the prepared helical PDA assemblies could serve as a direct visual probe for the enantioselective recognition of D - or L -lysine. The high enantioselectivity could be attributed to an inherent chiral recognition based on the steric repulsion of helical PDA assemblies towards the opposite chiral lysine. To confirm the above-mentioned hypothesis, X-ray diffraction (XRD) characterizations were performed for studying the packing structure changes of the samples associated with the chromatic transition. The sharp peaks observed in XRD analysis indicated the formation of a lamella structure. As for the left-handed helical PDA assemblies, after immersion in L -lysine solution for 2 h, the peak intensity dramatically decreased, indicating the partial destruction of the lamella packing structure, whereas no obvious change in XRD profiles could be detected for above left-handed helical PDA assemblies immersed into D -lysine solution (the same concentration) for 2 h ( Supplementary Fig. 11 ). All above results indicated that the interaction between left-handed helical PDA assemblies and L -lysine is stronger, leading to greater colour and spectral responses and the destruction of PDA assemblies. However, in the case of left-handed helical PDA assemblies and D -lysine, the interaction is weaker due to the steric repulsion, therefore no obvious colour or structural changes could be detected. Inspired by the preliminary results, we further investigated the enantioselectivity of the prepared helical PDA assemblies toward other chiral amino acids, as shown in Supplementary Fig. 12 . The prepared helical PDA assemblies exhibited enantioselective recognition behaviour toward arginine and histidine, however, no enantioselectivity or obvious colour change can be observed for alanine and glutamic acid ( Supplementary Fig. 13 ). Magnetochiral anisotropy has been suggested as an explanation for the homochirality of life [15] , [31] . Magnetochiral anisotropy may induce enantioselectivity in chemical reactions, however, few convincing demonstrations of such an effect have been observed. Previously, Rikken and Raupach showed that magnetochiral anisotropy could give rise to an enantiometric excess in a photochemical reaction driven by unpolarized light in a parallel magnetic field. The sample they used was chiral Cr(III) tris-oxalato complex, which is unstable in solution and exists as a racemic mixture and spontaneously dissociates and re-associates. On irradiation with unpolarized light in a parallel magnetic field, a small excess of one enantiomer is produced and maintained due to the enantiomeric excess photoresolution and spontaneous thermal racemization. As soon as the irradiation stops, the system will return to the racemic state owing to the thermal dissociation and random re-association of the complexes. However, it is not clear whether such magnetochiral anisotropy effect could be utilized into other photochemical reactions to produce chiral excess, especially from initially wholly achiral compound. Herein, we utilized the magnetochiral anisotropy to induce asymmetric photopolymerization reaction and realized the enantioselective synthesis of helical PDA assemblies from initially wholly achiral DA monomer for the first time. The significances of our study are twofold. First, we have realized the enantioselective synthesis of helical conjugated polymer from achiral monomer by the application of LPL irradiation in a parallel or antiparallel magnetic field. Our results show convincingly that magnetochiral anisotropy may induce enantioselectivity in photopolymerization reactions, even from initially wholly achiral monomer. Second, thus-formed helical PDA assemblies were stable and could be further used to distinguish the amino acid enantiomers through simple colorimetric methods. In summary, the asymmetric polymerization of disc-shaped DA derivative in the LC phase had been realized by application of LPL and the magnetic field based on magnetochiral dichroism mechanism. The screw direction of predominant helical PDA chain could be rigorously controlled with the relative orientation of LPL and the magnetic field. The helical PDA assemblies could serve as a direct visual probe for the discrimination of D - or L -lysine. This work not only provides responsive chromatic materials towards chiral recognition of amino acid enantiomers, but also is of great fundamental value for a deeper understanding of the mirror symmetry breaking in photochemical reaction through the magnetochiral dichroism effect. The preparation of the disc-shaped DA derivative 10, 12-Pentacosadiynoic acid was purchased from Tokyo Chemical Industry Co., Ltd., and purified before use. TTB was synthesized in analogy to the previous procedure [32] . HB complex was obtained by mixing TTB with 10, 12-Pentacosadiynoic acid in a 1:3 molar ratio in chloroform followed by slow evaporation of the solvent at reduced pressure. Then the disc-shaped mesogenic DA derivative could be achieved, in which three DA units were non-covalently linked to a C 3 -symmetric triazole derivative (TTB) core through HB interactions. The HB complex sample was firstly dissolved in CHCl 3 with a concentration of 10 mg ml −1 . Then films of DA monomers were prepared by spin-coating method. Polymerization of DA derivative Before polymerization, the films were heated to 47 °C to confirm that the disc-shaped DA derivative were in LC phase. Then, the above samples were polymerized by the application of LPL and the magnetic field, generated by an electromagnet, with the magnetic field parallel or antiparallel to the irradiation direction of LPL. The LPL (313±5 nm) was simply generated by using a combination of ultra-high pressure mercury lamp, a 313-nm interface filter and a UV polarizer. The light intensity could be switched from 0 to 20 mW cm −2 . How to cite this article: Xu, Y. et al. Enantioselective synthesis of helical polydiacetylene by application of linearly polarized light and magnetic field. Nat. Commun. 5:5050 doi: 10.1038/ncomms6050 (2014).